Natural gold particles inEucalyptusleaves and their relevance to exploration for buried gold deposits Eucalyptus trees may translocate Au from mineral deposits and support the use of vegetation (biogeochemical) sampling in mineral exploration, particularly where thick sediments dominate. However, biogeochemistry has not been routinely adopted partly because biotic mechanisms of Au migration are poorly understood. For example, although Au has been previously measured in plant samples, there has been doubt as to whether it was truly absorbed rather than merely adsorbed on the plant surface as aeolian contamination. Here we show the first evidence of particulate Au within natural specimens of living biological tissue (not from laboratory experimentation). This observation conclusively demonstrates active biogeochemical adsorption of Au and provides insight into its behaviour in natural samples. The confirmation of biogeochemical adsorption of Au, and of a link with abiotic processes, promotes confidence in an emerging technique that may lead to future exploration success and maintain continuity of supply. Mineral explorers need to find new ore deposits. New Au discoveries are down by 45% over the last 10 years [1] . Novel exploration techniques are required to find the more difficult deposits hidden beneath sediments [2] . Furthermore, these new techniques need to be underpinned by an improved understanding of mechanisms of metal mobilization that are currently poorly understood [3] . Biogeochemistry for mineral exploration is one such relatively new technique, but defining the boundaries as to when and where it may or may not be effective has been difficult [4] . One of the major technical problems facing research involving natural samples is that Au concentrations in vegetation are commonly very low (<1–2 p.p.b.) [5] , [6] . There is no unequivocal evidence that Au is actually absorbed by plants over mineral deposits and that currently measured Au is not merely a result of dust contamination of samples [7] , [8] . Thus explorers are reticent to embrace an important emerging technique in which they lack confidence in its applicability, data quality and interpretation of results. The Freddo Gold Prospect is an ideal location to investigate potential mechanisms for the chemical transport of Au. It is located 40 km north of Kalgoorlie (Western Australia) in the Yilgarn Craton and lies beneath a gently sloped drainage catchment with no known sources of surface contamination: It is undisturbed by mining activity, there is no outcropping mineral deposit and the Au itself is concealed by ~30 m of barren, Cainozoic alluvial and colluvial deposits infilling a palaeovalley ( Fig. 1 ) [9] . The mineral deposit at Freddo is a sub-economic supergene type measuring 100 m by 200 m at 35 m depth, discovered by exploratory drilling. The simplified regolith profile at Freddo consists (from top to bottom) of a red calcareous kaolinitic clay soil (2 m thick), grading to a mottled red and pale grey kaolinitic clay (12 m), grey smectitic clay (10 m), quartzose fluvial sand (8 m) overlying a saprolite of greenish brown smectitic clay containing Au ( Fig. 2 ). Fresh rock occurs at about 40 m depth. Large Eucalyptus trees (some >10 m in height) grow over the deposit in an open woodland setting and make it an ideal study site to examine the uptake of Au. 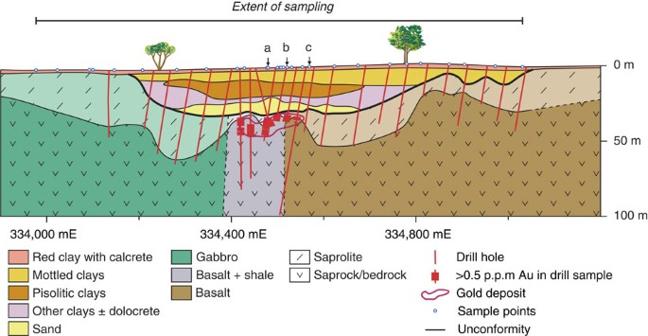Figure 1: Location of the sampling traverse at Freddo Au deposit. The underlying regolith stratigraphy and Au deposit is shown. The sampling traverse (1.3 km in length) is orientated perpendicular to the palaeochannel. Detailed sampling was undertaken at sites RD 50 (a), RD 56 (b) and RD 68 (c). Figure 1: Location of the sampling traverse at Freddo Au deposit. The underlying regolith stratigraphy and Au deposit is shown. The sampling traverse (1.3 km in length) is orientated perpendicular to the palaeochannel. Detailed sampling was undertaken at sites RD 50 ( a ), RD 56 ( b ) and RD 68 ( c ). 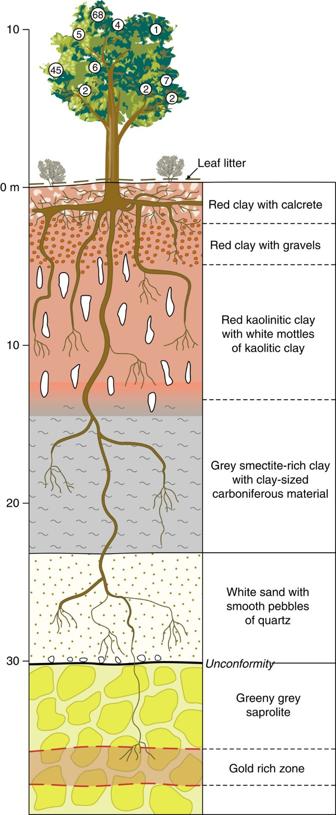Figure 2:Eucalyptusroot system through regolith at Freddo Au prospect. The relationship between theEucalyptusroot system, regolith stratigraphy and location of the Freddo Au deposit is shown. Circled numerical data in foliage corresponds to typical sample location and bulk Au analyses of leaves (seeSupplementary Fig. S1andSupplementary Table S2for samples RD50T1-1–10). Note the unconformity (marked by presence of rounded river pebbles) at 30 m depth beneath which is the weathered bedrock containing the Au deposit. Full size image Figure 2: Eucalyptus root system through regolith at Freddo Au prospect. The relationship between the Eucalyptus root system, regolith stratigraphy and location of the Freddo Au deposit is shown. Circled numerical data in foliage corresponds to typical sample location and bulk Au analyses of leaves (see Supplementary Fig. S1 and Supplementary Table S2 for samples RD50T1-1–10). Note the unconformity (marked by presence of rounded river pebbles) at 30 m depth beneath which is the weathered bedrock containing the Au deposit. Full size image At Barns Gold Prospect (25 km north of Wudinna, South Australia), previous studies have shown that vegetation samples, soil and calcrete have anomalously high Au contents [10] . Like Freddo, Barns is an undisturbed site well-suited to Au mobilization studies. The Barns Au deposit lies within Archean rocks of the Gawler Craton that have been weathered to 50 m depth [11] . The Barns regolith consists of saprolite overlain by up to 8 m high aeolian sand dunes that have developed over the last 20,000 years [10] . Gold is patchily distributed in the saprolite and there is a sub-economic Au supergene deposit (500 m by 200 m) 35 m below the dune. Calcrete within the top 2 m of the saprolite beneath the dune contains anomalous Au concentrations (35 p.p.b.) against a background of <1 p.p.b. Younger calcrete, intimately associated with plant roots (rhizoliths), occurs within the sand dune, and has an anomalous Au content (up to 9 p.p.b.) [10] . Small Eucalyptus trees (mostly <5 m in height) grow in the sand dunes over the deposit. The precipitation of nanoparticulate Au from laboratory studies, using a variety of biological, physiological and chemical procedures, are widely reported in the literature [12] and nanoparticulate Au has been documented in inorganic environments [13] . Greenhouse and laboratory experiments utilizing the uptake of Au by plants for nanoparticle production are frequently undertaken. These experiments typically use concentrations of Au much higher than that is found in the natural environment. However, there have been few reported greenhouse experiments undertaken to investigate Au uptake of plants commonly used in mineral exploration. Plants that have a natural barrier to Au uptake would negate their use in biogeochemical exploration [4] as the Au concentration in a plant would be unrelated to the Au concentration in the regolith in which it was growing. Here, native Australian Eucalyptus and Acacia seedlings were grown experimentally under greenhouse conditions in sand pots dosed with Au to investigate the location and nature of nanoparticles. We collect samples from two field sites (Freddo and Barns), conduct greenhouse experiments and complex analytical procedures to investigate the nature of Au variability and biotic–abiotic-linked mechanisms for Au mobilization and precipitation. A Eucalyptus tree investigated over the deeply buried Au deposit at Freddo has Au particles forming in its foliage with similar features to those grown in our laboratory experiments, whereas leaves at Barns demonstrate the release of Au-containing exudates. Collectively, these results are important for mineral explorers to consider as they access more difficult terrains with deeper sediments and assess more subtle surficial geochemical anomalies. Freddo Samples from the large (>10 m tall) Eucalyptus trees at Freddo were found to be highly anomalous in Au exclusively and directly over the buried deposit ( Fig. 3 , Supplementary Table S1 ). The maximum Au concentrations in dried leaves, twigs, bark, litter and soil were 80, 44, 4, 12 and 41 p.p.b., respectively, with background concentrations of 0.1 p.p.b. for plant material, 1 p.p.b. for litter and 6 p.p.b. for soil. Thus some tree parts (leaves and twigs) were richer in Au than others (bark). Tree trunk (heartwood and sapwood) samples contained between 0.1 and 0.7 p.p.b. Au. Owing to its large mass, the tree trunk represents a major storage organ for Au. 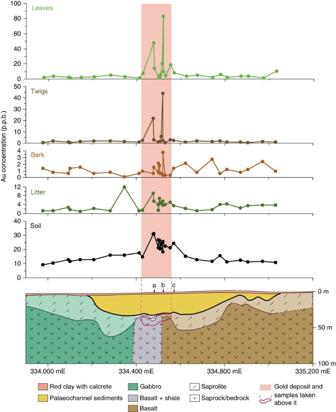Figure 3: Gold concentrations from sampling traverse at Freddo Au deposit. Data shows Au concentrations in parts per billion contained within a variety of sample media. A variety of sample media were tested for Au including bark, leaves, twigs and soil. Note how the concentrations of Au are highest in the leaves, twigs and soil sample media directly over the buried Au deposit (those highlighted in pink shading); litter and bark were not anomalous in Au. At sites RD 50 (a) and RD 68 (c), ten samples of foliage were taken from around the tree to examine the variability of Au in leaves (seeSupplementary Table S2). At site RD 56 (b), 20 leaves were taken from the reference bulk sample and Au variability was investigated in detail (seeSupplementary Table S3). Figure 3: Gold concentrations from sampling traverse at Freddo Au deposit. Data shows Au concentrations in parts per billion contained within a variety of sample media. A variety of sample media were tested for Au including bark, leaves, twigs and soil. Note how the concentrations of Au are highest in the leaves, twigs and soil sample media directly over the buried Au deposit (those highlighted in pink shading); litter and bark were not anomalous in Au. At sites RD 50 ( a ) and RD 68 ( c ), ten samples of foliage were taken from around the tree to examine the variability of Au in leaves (see Supplementary Table S2 ). At site RD 56 ( b ), 20 leaves were taken from the reference bulk sample and Au variability was investigated in detail (see Supplementary Table S3 ). Full size image In order to investigate the possibility of particulate Au in the Eucalyptus foliage, a three-stage sequential experimental procedure was adopted. First, ten foliage samples, consisting of leaves and twigs, were each collected from around the canopies of two trees, one over the deposit (RD50) and one over background, 200 m distant (RD68) (see Fig. 3 for location). Leaves (100 g sub-samples), separated from each of the ten foliage samples over the deposit, were analysed and had highly variable Au contents ranging from 1 to 68 p.p.b. (RD50) and 1 to 16 p.p.b. in background sample RD68 ( Supplementary Fig. S1 and Supplementary Table S2 ). Second, variable Au concentrations (5–359 p.p.b., mean 46 p.p.b. and standard deviation 64 p.p.b.) were noted again when 20 individual leaves were randomly selected from bulk sample RD56 (see Fig. 3 for location), divided into three leaf parts ( n =60) and separately analysed ( Supplementary Fig. S2 and Supplementary Table S3 ). Third, a further 20 leaves were randomly selected from bulk sample RD56. Sixty leaf discs (diameter of 6 mm) were punched out from the 20 leaves and analysed using the synchrotron X-ray Fluorescence Microprobe (XFM) equipped with a Maia detector [14] to maximize the probability of finding Au particles and to map the distribution of other elements ( Supplementary Figs S3 and S4 ). High-resolution (1 μm) mapping of the discs identified several Au particles up to 8 μm in length indicating that Au had precipitated naturally within the leaves ( Fig. 4a,b ). The XFM–Maia combination is particularly well-suited to penetrate organic matrices non-destructively, speedily map large areas at high resolution and detect small (1–10 μm) discrete heavy metal particles, for example, Au located within the matrix [15] . Some Au particles were associated with Ca oxalate crystals ( Fig. 4b ). This is the first time, to our knowledge, that naturally occurring (non-laboratory generated) Au particles have been imaged within the cells of biological tissue. Gold particles have been imaged adsorbed on the surface of tree bark but these probably have an aeolian origin [4] . 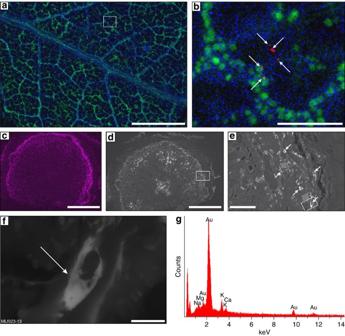Figure 4: Particulate Au and analytical data from laboratory-grown and natural specimens. (a) Synchrotron image showing distribution of Cu (blue), Sr (oxalate crystals, green) and Au (red) in natural leaf specimen. Strontium is a proxy for Ca; boxed area inais shown inb. (b) Detailed view showing isolated particulate Au grains (red, arrowed) and two of which are attached to the surface of Ca oxalate crystals (green). (c) SEM–EDS map of twig section showing examples of Au (purple) in laboratory-grown plants. (d) SEM BSE image of laboratory-grown plants incshowing plant structure with brighter areas showing Au; boxed area in (d) is shown ine. (e) Detailed BSE view showing distribution of Au (bright areas). Arrows point at some examples of Au (including those particles attached to Ca oxalate crystals); boxed area in (e) is shown inf. (f) Detailed BSE view showing Au particle 8 μm in length. (g) Spectra showing identification of Au by SEM–EDS. Scale bars ina,c,dandb,eandfindicate scale as 500, 50 and 5 μm, respectively. Figure 4: Particulate Au and analytical data from laboratory-grown and natural specimens. ( a ) Synchrotron image showing distribution of Cu (blue), Sr (oxalate crystals, green) and Au (red) in natural leaf specimen. Strontium is a proxy for Ca; boxed area in a is shown in b . ( b ) Detailed view showing isolated particulate Au grains (red, arrowed) and two of which are attached to the surface of Ca oxalate crystals (green). ( c ) SEM–EDS map of twig section showing examples of Au (purple) in laboratory-grown plants. ( d ) SEM BSE image of laboratory-grown plants in c showing plant structure with brighter areas showing Au; boxed area in ( d ) is shown in e . ( e ) Detailed BSE view showing distribution of Au (bright areas). Arrows point at some examples of Au (including those particles attached to Ca oxalate crystals); boxed area in ( e ) is shown in f . ( f ) Detailed BSE view showing Au particle 8 μm in length. ( g ) Spectra showing identification of Au by SEM–EDS. Scale bars in a , c , d and b , e and f indicate scale as 500, 50 and 5 μm, respectively. Full size image Samples taken from a soil profile near Freddo exemplify the strong relationship between Au and calcrete commonly found in southern Australia ( Fig. 5 ) [10] . Gold concentrations in the soil profile have a maximum of 177 p.p.b. and correspond to a concentration of 7.1% Ca (as calcite). The strong association between Ca and Au in the profile indicates that the physico-chemistry of these elements is controlled by a similar mechanism; where the Ca occurs as gypsum ( Fig. 5 ; Supplementary Table S4 ), the Au–Ca relationship is weaker. 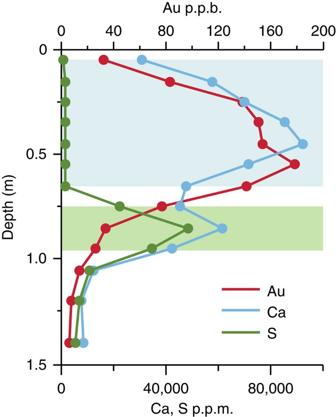Figure 5: Relationship between key elements in a calcareous soil profile near Freddo. The strong relationship between Au and Ca in the upper part of the profile (shaded blue, related to calcite) is common in Australian soils situated near Au deposits. The relationship between Au and Ca is weaker in the lower part of the profile as some of the Ca (with S) is in gypsum (shaded green) which is not associated with Au. Figure 5: Relationship between key elements in a calcareous soil profile near Freddo. The strong relationship between Au and Ca in the upper part of the profile (shaded blue, related to calcite) is common in Australian soils situated near Au deposits. The relationship between Au and Ca is weaker in the lower part of the profile as some of the Ca (with S) is in gypsum (shaded green) which is not associated with Au. Full size image Barns exudates Exudate samples collected from vegetation over the Barns deposit had 20 times more Au (maximum of 0.004 μg) than the background samples 800 m distant (0.0002 μg; Supplementary Fig. S5 and Supplementary Table S5 ). This indicates that Eucalyptus trees, in addition to compartmentalizing Au in Ca oxalate crystals (as found for the Freddo samples), expel soluble Au through their leaves. As exudates evaporate from the leaf surface Au salts are precipitated which, under normal circumstances, would be dislodged by wind or dissolved by rain and transferred to soil. Greenhouse study In a separate, related laboratory experiment, Eucalyptus and Acacia seedlings were grown experimentally under greenhouse conditions in sand pots and dosed with 1,000 p.p.m. Au. Scanning electron microscopy (SEM) (equipped with an energy-dispersive spectrometer (EDS)) analyses of the leaves showed that they contained Au particles with some partly coating Ca oxalate crystals in a similar manner to our observations in the natural samples ( Fig. 4c–g ). The demonstration of absorbed Au in vegetation in Eucalyptus foliage from Freddo and Barns is a crucial result in our understanding of Au mobilization. Identification of such naturally low concentrations of Au has not been attempted before but by carefully selecting samples (using the sequential procedure) with the highest concentration and using XFM–Maia, we maximized the probability of being able to achieve the observations. The larger natural Au particles appear to occur in an irregular shape similar to experimentally produced Au and, furthermore, the association of Au with Ca oxalate crystals was similar for natural and artificially produced specimens. Although Ca oxalate is principally involved with the regulation of Ca in the plant [16] , it has been implicated in toxic metal compartmentalization [17] . Gold is probably toxic to plants and is moved to its extremities [18] (such as leaves) or in preferential zones [19] within cells in order to reduce deleterious biochemical reactions. Gold toxicity is not confined to plants: recently, a biochemical mechanism for extracellular precipitation of Au by a bacterium was described [20] , [21] . The findings from these field sites and laboratory experiments enable us to propose a tentative model for Au mobilization and precipitation for this biotic–abiotic system. We assert that climatic and biological factors at Freddo, Barns and elsewhere are crucial for the transportation of Au to the surface from great depth. The Eucalyptus trees are part of woodland at Freddo and at Barns stretching over several thousand square kilometres. Both prospects are in semi-arid climates with annual average rainfall of 260–290 mm, evapotranspiration rates in excess of 2,600 mm per annum and average maximum January temperatures of 34 °C. Despite these harsh climatic conditions, it is significant that the large trees at Freddo, in particular, are able to thrive. The Eucalyptus root system is unusually deep and extensive [22] with sinker roots in one species ( Eucalyptus marginata ) documented at 40 m depth [23] ( Fig. 2 ) which, along with other physiological and anatomical adaptations, enables some species to flourish in an arid environment and be drought tolerant. For example, Eucalyptus species commonly have small, tough, vertically hanging leathery leaves comprised of hard sclerochyma tissue enabling them to resist wilting [24] . The link between abiotic and biotic geochemical processes at the earth surface is becoming demonstrably and irresistibly stronger. Our combined data indicate that there is a significant but irregularly distributed mass of Au within the tree derived from 35 m below the surface, which is released and accumulates in the soil after leaf fall and when the tree dies. Calcrete (pedogenic carbonate or caliche) is a common component of the soil in southern Australia and provides an inorganic testimony for this organic activity [25] . The phenomenon of Au accumulating in calcrete has been well documented, primarily in Australia [10] , [26] , [27] . Calcrete and Eucalyptus woodland growing in semi-arid areas of southern Australia are commonly associated [28] . Samples taken from the soil profile near Freddo illustrate the typical strong relationship between Au and calcrete in Eucalyptus woodland found elsewhere ( Fig. 5 ). The correlation between these two fundamentally different elements (Ca and Au) in calcrete is due to their similar physical response to rainfall and evapotranspiration (rather than a chemical response) averaged over thousands of years [10] . Calcrete is an evapotranspiration product, in part, of the trees rather than a specific adaptation by the trees to grow in alkaline soils [29] and is commonly intimately associated with plant roots, for example, as calcareous rhizoliths [30] . Calcrete’s calcite principally originates from inputs of meteoric (Ca, marine [31] ) and respiration (CO 2 , microbes and plant roots [32] ) origins. Soil moisture is required for Au and Ca to be mobilized and water-soluble (ionic) Au itself is nearly twice as high in calcrete (15%) compared with other near-surface regolith materials (8% (ref. 33 )). The Au association with calcrete has been widely exploited by the mineral exploration industry and many operating mines and prospects owe their existence to exploration targeting the Au in calcrete correlation [34] . Interestingly, most of these have been in Australia. Our preliminary model for the biomediated formation of abiotic and biotic Au anomalies in Eucalyptus woodland is tempered by climatic processes. Gold at the woodland surface (in plants and soil) is supplemented through deep-rooted trees that absorb and transport Au from the buried deposit. It is translocated to the trees from the deposit during times of high water demand when sinker roots access deeper regolith moisture [22] . Then, ionic Au is transported in water through the vascular system of the trees at sub-toxic concentrations then reduced (to Au 0 ) and precipitated within the cells of the tree. Gold occurs throughout the trees but the highest concentrations are found in the foliage where hydrostatic pressures fluctuate greatly. Gold crystals may grow as a result of the propensity of ionic Au to reduce and autocatalytically precipitate [35] . Gold is released from trees through leaf fall, leaf exudates, bark shedding, limb/branch loss and plant death and is transferred to soil. It may be dissolved in the soil and adsorbed through the lateral roots of understorey plants and trees. Plant debris (from trees and shrubs) contributes to degrading organic matter and creates subtle Au anomalies in the soil. Finally, Au is transported laterally and vertically in the soil (including those dominated by calcrete) through processes of physical erosion (litter and soil) and chemical dispersion [36] . Gold (and calcite) is precipitated with calcrete when moisture is removed by evapotranspiration but some is re-absorbed and precipitated in the plants. Micro-organisms [37] and fungi [38] are implicated in the mobilization and intra- and extra-cellular precipitation of Au in the rhizosphere. A dynamic equilibrium in the Au flux occurs for the soil-vegetation-deposit system although absolute concentrations in soil and plants are determined by other factors. For example, random dispersive environmental events such as wildfire, flood and strong winds serve to lower the flux so that Au brought to the surface by deep-rooted trees will no longer be able to sustain the soil Au concentrations at a sufficient rate to counteract erosional losses. We have considered alternative mechanisms of Au transport operating at depth, beneath cover but have found these to be unconvincing in these settings [2] . For example, the water tables at our study sites occur at about 30 m which reduces the possibility of transport of Au nanoparticles via gas bubbles [39] . The deposits are located within the tectonically stable Archean cratons and the paucity of recent tectonic activity to create faults suggests that seismic pumping of groundwater or barometric pumping of gases is unlikely to bring Au up to the trees [40] . Hydraulic lift by deep-rooted vegetation is a compelling mechanism of transport [41] . It not only provides an explanation for the Au adsorbed by the trees but also the existence of the Au in calcrete anomaly beneath them. Despite the decline in discoveries [1] , falling ore grades and increasing demand for Au [42] , new exploration technologies for Au deposits, incorporating the deep penetrating ability of certain trees, have been seldom reported [43] . Analytical problems, extremely low concentrations and variable data in comparison with traditional soil sampling have held back the use of vegetation for Au exploration [4] . Our results add to the mounting evidence that demonstrate enrichment of Au in biota and soils are inextricably linked and that disparity between biotic and abiotic processes at the Earth’s surface is, at best, indistinct [44] . Mineral exploration will benefit by embracing and understanding mechanisms of the biota-mineral-climate continuum and will be important in finding new Au deposits undercover into the future. General field sampling Soil samples (about 1 kg) were collected with a plastic trowel within 1 m of the base of the tree trunks and put into plastic bags. Sampling depth was from 0–10 cm. Bark samples (about 300 g) were collected from base of the tree trunk and placed into calico bags. Litter samples (about 300 g) were collected into calico bags from above where the soil sample was taken. Foliage (collected as branches, 2 kg) was removed from trees using Teflon-coated secateurs and a truck mounted cherry picker (or basket crane) at Freddo or from ground level at Barns. The leaves and twigs were separated from the main branches with Teflon-coated secateurs and placed into calico bags. All samples were collected during one campaign. Soil profile A soil profile was excavated using a back hoe excavator. The face of the soil profile was cleaned down with a brush and samples taken using a plastic trowel approximately every 0.1 m. Leaf exudates Dissolved leaf exudates were sampled and analysed from the foliage of Eucalyptus trees growing on the dunes using transpiration collectors ( Supplementary Fig. S6 ). Large plastic (transpiration) bags (1.2 m by 0.5 m) were placed around branches containing foliage (leaves and twigs). The opening of each bag was tied around the branches, supporting the foliage, using a plastic cable tie. A corner of the bag was tied to the trunk in such a way as to allow exudates to drain freely from the foliage into the bag. Bags were left tied around branches overnight for approximately 15 h after which time the plastic bag corner was cut and the exudates drained into a screw-capped plastic sample container. These were directly analysed by inductively coupled mass spectrometry (ICP-MS). Sample preparation For the foliage, leaves were separated from the branches in the laboratory to make the twig and leaf samples. The leaves, twigs, bark and litter were milled with a cross beater mill to a fine powder. Soil samples were sieved through a 250 μm plastic sieve and the sample milled to a nominal <75 μm particle size in a ring mill. General sample analyses About 10 g of organic-rich sample (that is, bark, litter, twigs and leaves) was submitted for analysis. Standards and duplicates analysed at the same time were in good agreement (errors <10%). About 4 g of material was digested with 10 ml of nitric acid overnight and then a further 10 ml of nitric and hydrochloric acids were added and digested for 2 h at 90 °C. The digest was diluted to a set volume and analysed by ICP-MS. For soil, about 25 g of sample was digested by aqua regia and analysed by ICP-MS. The X-ray diffraction was done using an Endeavour D4 (Bruker Corporation). The leaf parts (samples RD56T1-20 left, middle and right) were digested without milling using the procedure described above for organic samples and with smaller solution volumes to keep concentrations higher. The weight of individual leaf parts was recorded to calculate final concentration as dry weight. Greenhouse study Seeds of Eucalyptus salmonophloia and Acacia aneura were grown in 150 × 40 × 40 mm pots containing acid-washed beach sand and pelleted slow-release nutrient. The seedlings underwent four treatments (25 seedlings for each treatment) of Au solution: 0, 10, 100 and 1,000 p.p.b. Au. Gold was added daily (10 ml) in solution as a cyanide complex (KAuCN) dissolved in deionised water using a pipette. The experiment continued for 3 months. At the completion of this treatment one each of the Eucalyptus and Acacia plants of the grown plants from the 1,000 p.p.b. Au treatment had 10 ml of 1,000 p.p.m. Au added to them. Samples of these organic materials were mounted in epoxy resin and polished exposing the plant tissue ready for SEM analyses. Synchrotron analyses Leaf discs were punched out from the Freddo leaves using a 6 mm diameter tungsten steel hole punch. Three discs were punched from each of 20 leaves at random to make 60 samples. These were mounted directly on a Perspex holder using Mylar tape that was fixed, (in turn) in front of the beam source using locating magnets. The X-ray fluorescence analyses were performed with a Maia 384 detector array [45] at the Australian Synchrotron facility and X-rays focussed into a beam spot of ~1.5 μm, dwell of ~1–2 ms per pixel, energy of 16.5 KeV using the Kirkpatrick–Baez-mirror-based lens system on the X-ray Fluorescence Microprobe (XFM) beamline [15] . Platinum, Mn, Ni and Fe foils were used to calibrate the beam. This system enables rapid analysis (8 h) of a large area (~2 cm 2 ) at about 1–2 μm spatial resolution; this is at least an order of magnitude more efficient compared with conventional X-ray detectors to identify Au in soil samples. SEM analyses The SEM imaging and analyses were performed using a back-scattered electron (BSE) detector on a Philips XL40 controlled pressure SEM fitted with an energy-dispersive X-ray analysis EDS. How to cite this article: Lintern, M. et al. Natural gold particles in Eucalyptus leaves and their relevance to exploration for buried gold deposits. Nat. Commun. 4:2614 doi: 10.1038/ncomms3614 (2013).